Pair density wave at high magnetic fields in cuprates with charge and spin orders 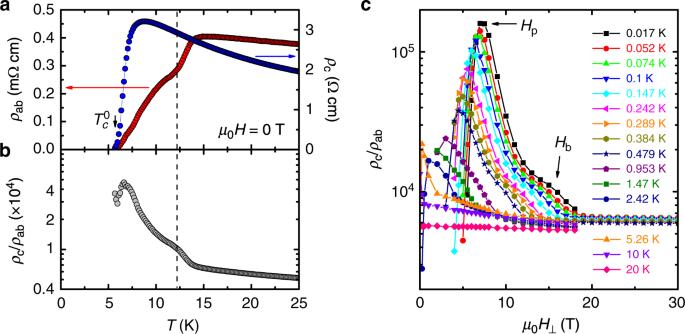Fig. 1: Evolution of the anisotropy in La1.7Eu0.2Sr0.1CuO4withTandH⊥. aρab(T) andρc(T), andbthe anisotropy ratioρc/ρab(T), in zero field. The vertical dashed line indicates where SC correlations are established in the planes, resulting in the enhancement of the anisotropy;ρccontinues to grow with decreasingT.cρc/ρabvs.H⊥at differentT, as shown. Arrows show the positions of the anisotropy peakHp, or the decoupling field, as well asHb, where the anisotropy is enhanced. The method to determineHbmore precisely is described in Supplementary Fig.1. In underdoped cuprates, the interplay of the pseudogap, superconductivity, and charge and spin ordering can give rise to exotic quantum states, including the pair density wave (PDW), in which the superconducting (SC) order parameter is oscillatory in space. However, the evidence for a PDW state remains inconclusive and its broader relevance to cuprate physics is an open question. To test the interlayer frustration, the crucial component of the PDW picture, we perform transport measurements on charge- and spin-stripe-ordered La 1.7 Eu 0.2 Sr 0.1 CuO 4 and La 1.48 Nd 0.4 Sr 0.12 CuO 4 in perpendicular magnetic fields ( H ⊥ ), and also with an additional field applied parallel to CuO 2 layers ( H ∥ ). We detect several phenomena predicted to arise from the existence of a PDW, including an enhancement of interlayer SC phase coherence with increasing H ∥ . These data also provide much-needed transport signatures of the PDW in the regime where superconductivity is destroyed by quantum phase fluctuations. The origin of the cuprate pseudogap regime has been a long-standing mystery. The richness of experimental observations [1] and the instability of underdoped cuprates towards a variety of ordering phenomena, such as periodic modulations of charge density discovered in all families of hole-doped cuprates [2] , have raised the possibility that putative pair density wave (PDW) correlations [3] , [4] may be responsible for the pseudogap regime [5] , [6] . In order to distinguish between different scenarios, the most intriguing open question is what happens at low \(T\ll {T}_{{\rm{c}}}^{0}\) (here \({T}_{{\rm{c}}}^{0}\) is the H = 0 superconducting (SC) transition temperature) and high H ⊥ , when SC order is destroyed by quantum phase fluctuations [6] and short-range charge orders are enhanced [7] , [8] , [9] . However, the experimental evidence for a PDW state remains scant and largely indirect in the first place. A PDW SC state was proposed [4] , [10] to explain the suppression of the interlayer ( c -axis) Josephson coupling (or dynamical layer decoupling) apparent in the H = 0 anisotropic transport [11] in La 1.875 Ba 0.125 CuO 4 , as well as in optical measurements in La 1.85− y Nd y Sr 0.15 CuO 4 when the Nd concentration was tuned into the stripe-ordered regime [12] . The dynamical layer decoupling was observed also in the presence of an applied H ⊥ , in La 1.905 Ba 0.095 CuO 4 (ref. [13] ) and La 2− x Sr x CuO 4 (ref. [14] ). In La 2− x − y (Ba,Sr) x (Nd,Eu) y CuO 4 compounds near x = 1/8, charge order appears in the form of stripes, which are separated by regions of oppositely phased antiferromagnetism (spin stripes) [5] at T < T SO < T CO ; here T SO and T CO are the onsets of spin and charge stripes, respectively. In La 2− x Sr x CuO 4 at x = 0.10, spin stripe order is induced [15] by applying H ⊥ . The dynamical layer decoupling was thus attributed [4] , [10] to a PDW SC state [3] , [10] , such that the spatially modulated SC order parameter, with zero mean, occurs most strongly within the charge stripes, but the phases between adjacent stripes are reversed (antiphase). Since stripes are rotated by 90° from one layer to next, antiphase superconductivity within a plane strongly frustrates the interlayer SC phase coherence [5] , leading to an increase in anisotropy. This effect is reduced by doping away from x = 1/8, but H ⊥ can lead to dynamical layer decoupling as static stripe order is stabilized by a magnetic field. To obtain more definitive evidence of the existence of a PDW, recent experiments have focused on testing various theoretical predictions [5] . For example, transport measurements on La 1.875 Ba 0.125 CuO 4 have employed H ⊥ high enough to decouple the planes and then to suppress the SC order within the planes, with the results consistent with pair correlations surviving in charge stripes [16] ; Josephson junction measurements [17] on La 1.875 Ba 0.125 CuO 4 devices support the prediction of a charge-4 e SC condensate, consistent with the presence of a PDW state; an additional charge order was detected [18] in Bi 2 Sr 2 CaCu 2 O 8 by scanning tunneling microscopy (STM) at very low \({H}_{\perp }/{T}_{{\rm{c}}}^{0}\,\lesssim \, 0.1\) T/K, consistent with a PDW order that emerges within the halo region surrounding a vortex core once a uniform SC order is sufficiently suppressed by H ⊥ . However, alternative explanations are still possible, and additional experiments are thus needed to search for a PDW and explore its interplay with other orders in the pseudogap regime [6] . Therefore, we measure transport in La 2− x − y Sr x (Nd,Eu) y CuO 4 compounds, which have the same low-temperature structure as La 2− x Ba x CuO 4 , over an unprecedented range of T down to \(T/{T}_{{\rm{c}}}^{0}\,\lesssim\, 0.003\) and fields up to \(H/{T}_{{\rm{c}}}^{0} \sim 10\) T/K. We combine linear in-plane resistivity ρ ab , nonlinear in-plane transport or voltage–current ( V – I ) characteristics, and the anisotropy ratio ρ c / ρ ab (here ρ c is the out-of-plane resistivity) to probe both charge and vortex matter on single crystals with the nominal composition La 1.7 Eu 0.2 Sr 0.1 CuO 4 and La 1.48 Nd 0.4 Sr 0.12 CuO 4 (see “Methods” section); the former is away from x = 1/8 and thus the stripe order is weaker [5] . We find signatures of dynamical layer decoupling in both H = 0 and with increasing H ⊥ , consistent with the presence of a PDW. However, a key proposed test of this interpretation involves relieving the interlayer frustration through the application of an in-plane magnetic field [5] , [10] . In particular, since H ∥ can reorient the spin stripes in every other plane [19] , [20] , [21] , a consequence of a PDW would be an enhancement of interplane coherence, or a reduced anisotropy. This is precisely what we test and observe. Anisotropy in H = 0 In both La 1.7 Eu 0.2 Sr 0.1 CuO 4 and La 1.48 Nd 0.4 Sr 0.12 CuO 4 , ρ c and ρ ab vanish at the same \({T}_{{\rm{c}}}^{0}\) within the error (see "Methods” section; see also Supplementary Note 1 ), indicating the onset of 3D superconductivity, similar to La 2− x Sr x CuO 4 (e.g. ref. [22] ). The initial drop of ρ ab ( T ) with decreasing T (Fig. 1 a) is accompanied by an enhancement of the anisotropy (Fig. 1 b), which continues to increase by almost an order of magnitude as T is lowered further towards \({T}_{{\rm{c}}}^{0}\) . These data look remarkably similar to those on La 1.875 Ba 0.125 CuO 4 (ref. [11] ) that motivated theoretical proposals for a PDW SC state in striped cuprates: the initial, high- T enhancement of the anisotropy is understood to reflect the establishment of SC correlations in CuO 2 planes. Fig. 1: Evolution of the anisotropy in La 1.7 Eu 0.2 Sr 0.1 CuO 4 with T and H ⊥ . a ρ ab ( T ) and ρ c ( T ), and b the anisotropy ratio ρ c / ρ ab ( T ), in zero field. The vertical dashed line indicates where SC correlations are established in the planes, resulting in the enhancement of the anisotropy; ρ c continues to grow with decreasing T . c ρ c / ρ ab vs. H ⊥ at different T , as shown. Arrows show the positions of the anisotropy peak H p , or the decoupling field, as well as H b , where the anisotropy is enhanced. The method to determine H b more precisely is described in Supplementary Fig. 1 . Full size image Evolution of the anisotropy and ρ ab with H ⊥ and T The evolution of ρ c / ρ ab ( T ) with H ⊥ is shown in Fig. 1 c. The anisotropy at the highest T = 20 K is ρ c / ρ ab ~ 6000 and practically independent of H ⊥ . However, as T is lowered below \({T}_{{\rm{c}}}^{0}\) , ρ c / ρ ab develops a distinctly nonmonotonic behavior as a function of H ⊥ . At T = 0.017 K, for example, the anisotropy increases with H ⊥ by over an order of magnitude before reaching a peak ( ρ c / ρ ab > 10 5 ) at H ⊥ = H p , signifying decoupling of or the loss of phase coherence between the planes. However, strong SC correlations persist in the planes for H ⊥ > H p : here ρ c / ρ ab decreases with H ⊥ to H ⊥ -independent values, comparable to those at high T , for the highest H ⊥ > 20 T. This is in agreement with previous evidence [23] that the H ⊥ > 20 T region corresponds to the normal state. A smooth, rapid decrease of the anisotropy for H ⊥ > H p is interrupted by a bump or an enhancement in ρ c / ρ ab , centered at H b . Therefore, the behavior of ρ c / ρ ab is qualitatively the same whether the SC transition is approached from either (1) the high- T normal state by lowering T in H = 0 (Fig. 1 b) or (2) the high- H ⊥ normal state by reducing H ⊥ at a fixed T (Fig. 1 c). These results thus suggest that the enhancement of the anisotropy near H b ( T ) may be attributed to the establishment of SC correlations in the planes as the SC transition is approached from the high-field normal state. This picture is supported by the comparison of ρ c / ρ ab , as a function of T and H ⊥ , with the behavior of ρ ab ( T ) for a fixed H ⊥ , as shown in Fig. 2 for both La 1.7 Eu 0.2 Sr 0.1 CuO 4 and La 1.48 Nd 0.4 Sr 0.12 CuO 4 . The ρ ab ( T ) data were extracted from the in-plane magnetoresistance (MR) measurements (ref. [23] , Supplementary Fig. 2 a; unless stated otherwise, the results are shown for La 1.7 Eu 0.2 Sr 0.1 CuO 4 sample B, see “Methods” section); the raw ρ c ( H ) data are shown in Supplementary Fig. 2 b, c. In Fig. 2 a, b, we also include T c ( H ⊥ ), as well as H peak , the position of the peak in the in-plane MR (see e.g. Supplementary Fig. 2 a), which corresponds [23] to the upper critical field H c2 in these materials (see also Supplementary Note 1 ). Indeed, at a fixed T , ρ c / ρ ab starts to increase as H ⊥ is reduced below H peak . This is followed by an enhancement of ρ c / ρ ab near H ⊥ = H b , corresponding to the initial, metallic-like drop of ρ ab ( T ) as the SC transition is approached from the normal state for a fixed H ⊥ (Fig. 2 c, d). The behavior of both materials is similar, except that the layer decoupling field H p ( T ) ≳ H c ( T ) [or T c ( H ⊥ )] in La 1.48 Nd 0.4 Sr 0.12 CuO 4 , as expected [5] for a stronger stripe order and frustration of interlayer coupling for x ≈ 1/8. Therefore, practically all the data in Fig. 2 c, d, i.e. for H ⊥ > H p , involve “purely” 2D physics, with no communication between the planes. The striking splitting of the ρ ab ( T ) curves in both materials (ref. [23] , Fig. 2 c, d), into either metallic-like (i.e. SC-like) or insulating-like, when the normal state sheet resistance R □/layer ≈ R Q , where R Q = h /(2 e ) 2 is the quantum resistance for Cooper pairs, further supports this conclusion: it agrees with the expectations for a 2D superconductor–insulator transition (SIT) driven by quantum fluctuations of the SC phase [24] . In addition, as previously noted [23] , the two-step ρ ab ( T ) is reminiscent of that in granular films of conventional superconductors and systems with nanoscale phase separation, including engineered Josephson junction arrays, where they are generally attributed to the onset of local (e.g. in islands or puddles) and global, 2D superconductivity. Similarities to the behavior of various SC 2D systems [25] , [26] thus suggest the formation of SC islands as H ⊥ is reduced below H b at a fixed T (e.g. Fig. 2 a, b), i.e. 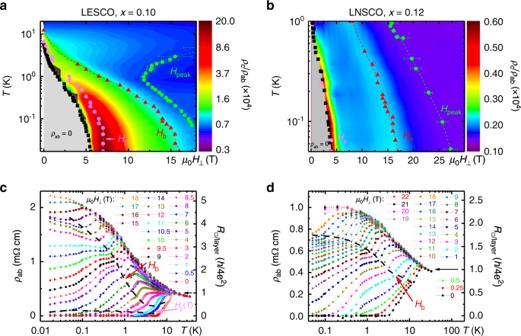Fig. 2: Anisotropy and the in-plane resistivity for differentTandH⊥. The color map inaandbshowsρc/ρabin La1.8−xEu0.2SrxCuO4(LESCO) withx= 0.10 (data from Fig.1c) and La1.6−xNd0.4SrxCuO4(LNSCO) withx= 0.12, respectively. Black squares:Tc(H⊥);ρab= 0 for allT<Tc(H⊥). Green dots:Hpeak(T), i.e. fields above which the in-plane MR changes from positive to negative; it has been established23thatHpeak(T) ~Hc2(T), i.e. the upper critical field. The error bars reflect the uncertainty in defining the MR peak within our experimental resolution (see inset of Supplementary Fig.2a for an example; also see Supplementary Fig.6a and ref.23for the raw MR data). Pink dots:Hp(T), the layer decoupling field; red triangles:Hb(T), where SC correlations are established in the planes as the SC transition is approached from the normal state.ρab(T) ofcLa1.7Eu0.2Sr0.1CuO4anddLa1.48Nd0.4Sr0.12CuO4for severalH⊥, as shown. Open symbols incshow the data from another run. Short-dashed lines guide the eye. TheHb(T) values obtained from the anisotropy are represented by the black dashed lines, as shown. The lower black dashed line inccorresponds to the layer decoupling field,Hp(T). Ind,Hp(T)≳Hc(T) [orTc(H⊥)]. Black arrows incanddshow that the splitting of theρab(T) curves for differentH⊥becomes pronounced whenR□/layer≈RQ=h/(2e)2. at the initial, metallic-like drop of ρ ab ( T ) for a fixed H ⊥ ( H b dashed line in Fig. 2 c, d). Additional evidence in support of this interpretation, such as the V – I that is characteristic of a viscous vortex liquid in the puddle regime, is discussed in Supplementary Note 2 (also, Supplementary Figs. 3 – 5 ). Therefore, at low T , the increasing H ⊥ destroys the superconductivity in the planes by quantum phase fluctuations of Josephson-coupled SC puddles. The evolution of this puddle region with T can be traced to the initial, metallic-like drop of ρ ab ( T ) at \(T\,> \,{T}_{{\rm{c}}}^{0}\) in H = 0 (see H b dashed line in Fig. 2 c, d, and Supplementary Figs. 3 and 4 ). Further increase of H ⊥ at low T then leads to the loss of SC phase coherence in individual puddles and, eventually, transition to the high-field normal state. These results are summarized in the sketch of the phase diagram, shown in Fig. 3 a. Fig. 2: Anisotropy and the in-plane resistivity for different T and H ⊥ . The color map in a and b shows ρ c / ρ ab in La 1.8− x Eu 0.2 Sr x CuO 4 (LESCO) with x = 0.10 (data from Fig. 1 c) and La 1.6− x Nd 0.4 Sr x CuO 4 (LNSCO) with x = 0.12, respectively. Black squares: T c ( H ⊥ ); ρ ab = 0 for all T < T c ( H ⊥ ). Green dots: H peak ( T ), i.e. fields above which the in-plane MR changes from positive to negative; it has been established [23] that H peak ( T ) ~ H c2 ( T ), i.e. the upper critical field. The error bars reflect the uncertainty in defining the MR peak within our experimental resolution (see inset of Supplementary Fig. 2 a for an example; also see Supplementary Fig. 6 a and ref. [23] for the raw MR data). Pink dots: H p ( T ), the layer decoupling field; red triangles: H b ( T ), where SC correlations are established in the planes as the SC transition is approached from the normal state. ρ ab ( T ) of c La 1.7 Eu 0.2 Sr 0.1 CuO 4 and d La 1.48 Nd 0.4 Sr 0.12 CuO 4 for several H ⊥ , as shown. Open symbols in c show the data from another run. Short-dashed lines guide the eye. The H b ( T ) values obtained from the anisotropy are represented by the black dashed lines, as shown. The lower black dashed line in c corresponds to the layer decoupling field, H p ( T ). In d , H p ( T ) ≳ H c ( T ) [or T c ( H ⊥ )]. Black arrows in c and d show that the splitting of the ρ ab ( T ) curves for different H ⊥ becomes pronounced when R □/layer ≈ R Q = h /(2 e ) 2 . Full size image Fig. 3: Evidence for a PDW from anisotropic transport . a Schematic T – H ⊥ phase diagram. H ⊥ suppresses the 3D superconductivity (gray) and decouples (dotted line) the CuO 2 layers at H ⊥ = H p ( T ). Strong SC phase fluctuations persist in the planes up to H c2 ( T ) (short-dashed line). The behavior in the pink region, the precursors of which appear already in H = 0 at \(T\,> \,{T}_{{\rm{c}}}^{0}\) (see dashed lines), is consistent with the presence of SC puddles in CuO 2 planes. An additional, in-plane field enhances the interlayer coupling for H p ( T ) < H ⊥ < H c2 ( T ), consistent with the presence of PDW correlations (thin hatched lines). Except for the thick solid line, other lines do not represent phase boundaries, but correspond to finite-temperature crossovers. b ρ c / ρ ab (for La 1.7 Eu 0.2 Sr 0.1 CuO 4 in-plane sample B1) vs. H ⊥ for different H ∥ , as shown, at T = 0.070 K. Larger inset: Enlarged view of the same data shows the suppression of the anisotropy by H ∥ for H p < H ⊥ < H c2 . Smaller inset: ρ c / ρ ab is reduced by  ~10% near H p by H ∥ up to 10 T. c The corresponding [ ρ ab ( H ∥ )/ ρ ab ( H ∥ = 0) − 1] (top, sample B1) and [ ρ c ( H ∥ )/ ρ c ( H ∥ = 0) − 1] (bottom) vs. H ⊥ at T = 0.028 K for different H ∥ , as shown. In all panels, solid lines guide the eye. Full size image Our experiments are thus consistent with the presence of local PDW correlations (in puddles) at \(T\,> \,{T}_{{\rm{c}}}^{0}\) in H = 0, which are overtaken by the uniform d-wave superconductivity at low \(T\,<\,{T}_{{\rm{c}}}^{0}\) . In transport, the PDW SC order becomes apparent when the uniform d-wave order is sufficiently weakened by H ⊥ : it appears beyond the melting field of the vortex solid, within the vortex liquid regime, i.e. in the regime of strong 2D phase fluctuations. Higher fields H p are needed to decouple the layers in La 1.7 Eu 0.2 Sr 0.1 CuO 4 than in La 1.48 Nd 0.4 Sr 0.12 CuO 4 , since it is farther away from x = 1/8. In the T → 0 limit and for even higher H ⊥ (< H c2 ), the system seems to break up into SC puddles with the PDW order. However, the final and key test of the presence of a PDW requires the application of a suitable perturbation, in particular H ∥ , to reduce the interlayer frustration and decrease the anisotropy [5] . Effects of H ∥ on the anisotropy We have performed angle-dependent measurements of both ρ ab ( H ) and ρ c ( H ), where the angle θ is between H and the crystalline c -axis. This has allowed us to explore the effect of in-plane fields \({H}_{\parallel }=H\sin \theta\) at different \({H}_{\perp }=H\cos \theta\) , i.e. fields parallel to the c -axis, discussed above. The angle-dependent ρ ab ( H ) was measured also on another La 1.7 Eu 0.2 Sr 0.1 CuO 4 sample (sample B1, see “Methods” section; Supplementary Fig. 8 ); the results are qualitatively the same on both samples. 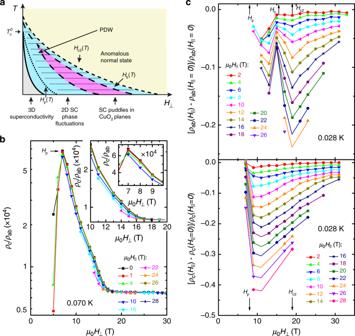Fig. 3:Evidence for a PDW from anisotropic transport. aSchematicT–H⊥phase diagram.H⊥suppresses the 3D superconductivity (gray) and decouples (dotted line) the CuO2layers atH⊥=Hp(T). Strong SC phase fluctuations persist in the planes up toHc2(T) (short-dashed line). The behavior in the pink region, the precursors of which appear already inH= 0 at\(T\,> \,{T}_{{\rm{c}}}^{0}\)(see dashed lines), is consistent with the presence of SC puddles in CuO2planes. An additional, in-plane field enhances the interlayer coupling forHp(T) <H⊥<Hc2(T), consistent with the presence of PDW correlations (thin hatched lines). Except for the thick solid line, other lines do not represent phase boundaries, but correspond to finite-temperature crossovers.bρc/ρab(for La1.7Eu0.2Sr0.1CuO4in-plane sample B1) vs.H⊥for differentH∥, as shown, atT= 0.070 K. Larger inset: Enlarged view of the same data shows the suppression of the anisotropy byH∥forHp<H⊥<Hc2. Smaller inset:ρc/ρabis reduced by  ~10% nearHpbyH∥up to 10 T.cThe corresponding [ρab(H∥)/ρab(H∥= 0) − 1] (top, sample B1) and [ρc(H∥)/ρc(H∥= 0) − 1] (bottom) vs.H⊥atT= 0.028 K for differentH∥, as shown. In all panels, solid lines guide the eye. Figure 3 b illustrates the effect of H ∥ on ρ c / ρ ab at low T = 0.070 K on sample B1 (see Supplementary Fig. 9 a–d for the raw ρ c and ρ ab data at different T ). Clearly, there is no effect of H ∥ for H ⊥ > H c2 ( T = 0.070 K) ≈ 17.5 T. Since H ∥ should break up Cooper pairs through the Zeeman effect, this confirms the absence of any observable remnants of superconductivity above the previously identified [23] H c2 (along c -axis). In contrast, for H p ≤ H ⊥ < H c2 , H ∥ reduces the anisotropy, which is precisely what is expected in the presence of a PDW SC state if the dominant effect of H ∥ is to reorient the spin stripes [10] . To understand exactly how H ∥ affects the anisotropy, we also investigate Δ ρ ab = ρ ab ( H ∥ ) − ρ ab ( H ∥ = 0) and Δ ρ c = ρ c ( H ∥ ) − ρ c ( H ∥ = 0) at different H ⊥ (Fig. 3 c and Supplementary Fig. 8 d for sample B1; Supplementary Fig. 9 e–h for sample B). It is obvious that ρ ab is reduced by H ∥ for all H ⊥ , which is the opposite of what would be expected if pair-breaking was dominant. The suppression of ρ ab is weaker for those H ⊥ where the superconductivity is stronger, e.g. near H b ~ 15 T in Fig. 3 c, and conversely, it is most pronounced above H c2 , indicating that the dominant effect of H ∥ is not related to superconductivity. In fact, it occurs most strongly in the two regimes where ρ ab ( H ⊥ ) exhibits hysteretic behavior at low T (Supplementary Figs. 3 and 6 ); the latter is attributed to the presence of domains with spin stripes (see also Supplementary Note 2 and Supplementary Fig. 7 ). This observation, therefore, further supports the conclusion that the main effect of H ∥ is the reorientation of spin stripes in every other plane [19] , [20] , [21] (see also Supplementary Note 3 ). The suppression of ρ ab by H ∥ seems to vanish at experimentally inaccessible H ⊥ , where the anomalous, insulating-like \(\mathrm{ln}\,(1/T)\) dependence observed in the field-induced normal state also appears to vanish [23] , suggesting that the origin of the \(\mathrm{ln}\,(1/T)\) behavior might be related to the presence of short-range spin stripes. As the spin stripes in every other plane are rotated by H ∥ , in the PDW picture the interlayer frustration should be suppressed, leading to a decrease in ρ c . This is precisely what is observed (Fig. 3 c). The anisotropy ratio ρ c / ρ ab is reduced (Fig. 3 b) because the effect of H ∥ on ρ c is relatively stronger than on ρ ab . Similar results are obtained in La 1.48 Nd 0.4 Sr 0.12 CuO 4 (Supplementary Fig. 10 ): here the reduction in ρ c is weaker than in La 1.7 Eu 0.2 Sr 0.1 CuO 4 and ρ ab is not affected within the experimental resolution, both consistent with the stronger pinning of stripe order at x = 1/8 (see also Supplementary Note 3 ). Nevertheless, the reduction of ρ c / ρ ab by H ∥ is comparable to that in La 1.7 Eu 0.2 Sr 0.1 CuO 4 (Fig. 3 b). Therefore, by applying an in-plane magnetic field, as proposed theoretically [5] , [10] , our measurements confirm the presence of a PDW in both La 1.7 Eu 0.2 Sr 0.1 CuO 4 and La 1.48 Nd 0.4 Sr 0.12 CuO 4 . The effects of H ∥ are observable up to \(T\,> \,{T}_{{\rm{c}}}^{0}\) (i.e. T ~ T SO in La 1.7 Eu 0.2 Sr 0.1 CuO 4 : Supplementary Fig. 9 ), providing additional evidence for the PDW correlations in H = 0 at \(T\,> \,{T}_{{\rm{c}}}^{0}\) , as sketched in Fig. 3 a. Our findings are thus consistent with the presence of local, PDW pairing correlations that compete with the uniform SC order at \({T}_{{\rm{c}}}^{0}\,<\,T\,<\,(2-6){T}_{{\rm{c}}}^{0}\) , and become dominant at intermediate H ⊥ as T → 0. Our results also provide an explanation for the surprising, and a priori counterintuitive, observation [23] that H c2 in La 1.48 Nd 0.4 Sr 0.12 CuO 4 ( H c2 ~ 25 T) is higher than that in La 1.7 Eu 0.2 Sr 0.1 CuO 4 ( H c2 ~ 20 T), even though its zero-field \({T}_{{\rm{c}}}^{0}\) is lower because of stronger stripe correlations. It is clear, though, that it is precisely because of the stronger stripe order and the presence of a more robust PDW SC state at x ≈ 1/8 that the superconductivity persists to higher fields as T → 0. In summary, by probing the previously inaccessible high \({H}_{\perp }/{T}_{{\rm{c}}}^{0}\) and T → 0 regime dominated by quantum phase fluctuations and by testing a theoretical prediction, we have obtained evidence consistent with the existence of a PDW state in the La-214 family of cuprates with stripes. Our observation of several signatures of a PDW in the regime with many vortices (i.e. a vortex liquid) is also consistent with the STM evidence [18] for a PDW order that emerges in vortex halos. Since the observed PDW correlations extend only up to T ≪ T pseudogap and not beyond H c2 ( T ), our results do not support a scenario in which the PDW correlations are responsible for the pseudogap. Samples Several single crystal samples of La 1.8− x Eu 0.2 Sr x CuO 4 with a nominal x = 0.10 and La 1.6− x Nd 0.4 Sr x CuO 4 with a nominal x = 0.12 were grown by the traveling-solvent floating-zone technique [27] . The high homogeneity of the crystals was confirmed by several techniques, as discussed in detail elsewhere [23] . It was established that the samples were at least as homogeneous as those previously reported in the literature and, in fact, the disorder in our La 1.7 Eu 0.2 Sr 0.1 CuO 4 crystals was significantly lower than that in other studies. We note that the trivial possibility that the two-step SC transition observed at H = 0 (e.g. Fig. 2 c, d for La 1.7 Eu 0.2 Sr 0.1 CuO 4 and La 1.48 Nd 0.4 Sr 0.12 CuO 4 , respectively) may be due to an extrinsic inhomogeneity, e.g. the presence of two regions with different values of \({T}_{{\rm{c}}}^{0}\) , is clearly ruled out also by the behavior of d ρ ab /d T with H ⊥ (Supplementary Figs. 3 a, 4 , and 8 b). In particular, both materials exhibit a reentrant metallic-like behavior at high H ⊥ , below H c2 (e.g. see the reentrant darker blue color band for La 1.48 Nd 0.4 Sr 0.12 CuO 4 ). This is the opposite of what is expected in case of two different \({T}_{{\rm{c}}}^{0}\) values corresponding to different doping levels, where one would expect a gradual suppression of superconductivity with H ⊥ , i.e. no reentrance. The samples were shaped as rectangular bars suitable for direct measurements of the in-plane and out-of-plane resistance. In La 1.7 Eu 0.2 Sr 0.1 CuO 4 , detailed measurements of ρ ab were performed on sample B with dimensions 3.06 × 0.53 × 0.37 mm 3 ( a × b × c ); ρ c was measured on a bar with 0.34 × 0.41 × 1.67 mm 3 . The in-plane La 1.48 Nd 0.4 Sr 0.12 CuO 4 crystal with dimensions 3.82 × 1.19 × 0.49 mm 3 was cut along the crystallographic [110] and [1 \(\bar{1}\) 0] axes, i.e. at a 45° angle with respect to a and b . A bar with 0.21 × 0.49 × 3.9 mm 3 ( a × b × c ) was used to measure ρ c in La 1.48 Nd 0.4 Sr 0.12 CuO 4 . The behavior of these samples remained stable for the duration of numerous experimental runs carried out in different cryostats and magnets (see below) that were needed for this study. After  ~3 years, the low- T properties of sample B changed, resulting in a quantitatively different T – H ⊥ phase diagram (Supplementary Fig. 8 b); this is why we consider it a different sample (B1). The phase diagram of sample B1 seems to be intermediate to those of sample B (Supplementary Fig. 3 a) and La 1.48 Nd 0.4 Sr 0.12 CuO 4 (Supplementary Fig. 4 ). Electrical contacts were made by evaporating Au on polished crystal surfaces such that, for current contacts, the two opposing faces were fully covered with Au to ensure a uniform current flow, while multiple voltage contacts made on the side faces were narrow enough to minimize the error in the absolute values of the resistance. This was followed by annealing in air at 700 °C. The data are shown for the voltage contacts separated by 1.53 mm for La 1.7 Eu 0.2 Sr 0.1 CuO 4 and 2.00 mm for La 1.48 Nd 0.4 Sr 0.12 CuO 4 in-plane samples; 0.47 mm for La 1.7 Eu 0.2 Sr 0.1 CuO 4 and 1.26 mm for La 1.48 Nd 0.4 Sr 0.12 CuO 4 out-of-plane samples. Dupont 6838 Ag paste was used to attach gold leads (≈25 μm thick) to the samples, with a subsequent heat treatment at 450 °C in the flow of oxygen for 15 min. The room T contact resistances were <0.1 Ω for La 1.7 Eu 0.2 Sr 0.1 CuO 4 , i.e. <0.5 Ω for La 1.48 Nd 0.4 Sr 0.12 CuO 4 . The properties of the samples, including the values of \({T}_{{\rm{c}}}^{0}\) , did not depend on the choice of voltage contacts used in the measurements, as expected in the absence of extrinsic (i.e. compositional) inhomogeneity. \({T}_{{\rm{c}}}^{0}\) was defined as the temperature at which the linear resistivity becomes zero, i.e. falls below the experimental noise floor (~0.5 mΩ). For the in-plane samples, \({T}_{{\rm{c}}}^{0}=(5.7\pm 0.3)\) K for La 1.7 Eu 0.2 Sr 0.1 CuO 4 and \({T}_{{\rm{c}}}^{0}=(3.6\pm 0.4)\) K for La 1.48 Nd 0.4 Sr 0.12 CuO 4 ; the out-of-plane resistivity ρ c vanishes at (5.5 ± 0.3) K for La 1.7 Eu 0.2 Sr 0.1 CuO 4 and (3.4 ± 0.5) K for La 1.48 Nd 0.4 Sr 0.12 CuO 4 . In La 1.7 Eu 0.2 Sr 0.1 CuO 4 , T SO ~ 15 K, T CO ~ 40 K (ref. [28] ), and the pseudogap temperature T pseudogap ~ 175 K (ref. [29] ); in La 1.48 Nd 0.4 Sr 0.12 CuO 4 , T SO ~ 50 K, T CO ~ 70 K (ref. [30] ), and T pseudogap ~ 150 K (ref. [29] ). Measurements The standard four-probe ac method (~13 Hz) was used for measurements of the sample resistance, with the excitation current (density) of 10 μA (~5 × 10 −3 and  ~2 × 10 −3 A cm −2 for La 1.7 Eu 0.2 Sr 0.1 CuO 4 and La 1.48 Nd 0.4 Sr 0.12 CuO 4 , respectively) for the in-plane samples and 10 nA (~7 × 10 −6 and ≲ 10 −5 A cm −2 for La 1.7 Eu 0.2 Sr 0.1 CuO 4 and La 1.48 Nd 0.4 Sr 0.12 CuO 4 , respectively) for the out-of-plane samples. d V /d I measurements were performed by applying a dc current bias (density) down to 2 μA (~1 × 10 −3 and  ~4 × 10 −4 A cm −2 for La 1.7 Eu 0.2 Sr 0.1 CuO 4 and La 1.48 Nd 0.4 Sr 0.12 CuO 4 in-plane samples, respectively) and a small ac current excitation I ac ≈ 1 μA (~13 Hz) through the sample and measuring the ac voltage across the sample. For each value of I dc , the ac voltage was monitored for 300 s and the average value recorded. The relaxations of d V /d I with time, similar to that in Supplementary Fig. 7 , were observed only at the lowest T ~ 0.016 K. Even then, the change of d V /d I during the relaxation, reflected in the error bars for the T = 0.017 K data in Supplementary Fig. 3 c, was much smaller than the change of d V /d I with I dc . The data that were affected by Joule heating at large dc bias were not considered. To reduce the noise and heating by radiation in all measurements, a 1 kΩ resistor in series with a π filter [5 dB (60 dB) noise reduction at 10 MHz (1 GHz)] was placed in each wire at the room temperature end of the cryostat. The experiments were conducted in several different magnets at the National High Magnetic Field Laboratory: a dilution refrigerator (0.016 K ≤ T ≤ 0.7 K) and a 3 He system (0.3 K ≤ T ≤ 35 K) in superconducting magnets ( H up to 18 T), using 0.1–0.2 T min −1 sweep rates; a portable dilution refrigerator (0.02 K ≤ T ≤ 0.7 K) in a 35 T resistive magnet, using 1 T min −1 sweep rate; and a 3 He system (0.3 K ≤ T ≤ 20 K) in a 31 T resistive magnet, using 1–2 T min −1 sweep rates. Below  ~0.06 K, it was not possible to achieve sufficient cooling of the electronic degrees of freedom to the bath temperature, a common difficulty with electrical measurements in the mK range. This results in a slight weakening of the ρ ab ( T ) curves below  ~0.06 K for all fields. We note that this does not make any qualitative difference to the phase diagram (Supplementary Fig. 3 a). The fields were swept at constant temperatures, and the sweep rates were low enough to avoid eddy current heating of the samples. The MR measurements with H ∥ c were performed also by reversing the direction of H to eliminate by summation any Hall effect contribution to the resistivity. Moreover, since Hall effect had not been explored in these materials in large parts of the phase diagrams studied here, we have also carried out detailed measurements of the Hall effect; the results of that study will be presented elsewhere [31] . The resistance per square per CuO 2 layer R □/layer = ρ ab / l , where l = 6.6 Å  is the thickness of each layer.